Supporting conditional mouse mutagenesis with a comprehensive cre characterization resource Full realization of the value of the loxP -flanked alleles generated by the International Knockout Mouse Consortium will require a large set of well-characterized cre-driver lines. However, many cre driver lines display excision activity beyond the intended tissue or cell type, and these data are frequently unavailable to the potential user. Here we describe a high-throughput pipeline to extend characterization of cre driver lines to document excision activity in a wide range of tissues at multiple time points and disseminate these data to the scientific community. Our results show that the majority of cre strains exhibit some degree of unreported recombinase activity. In addition, we observe frequent mosaicism, inconsistent activity and parent-of-origin effects. Together, these results highlight the importance of deep characterization of cre strains, and provide the scientific community with a critical resource for cre strain information. Conditional gene targeting, which allows for the spatial and temporal control of genetic modifications, has contributed to the significant increase in the number, diversity and availability of genetically engineered mice. One such system, cre- loxP , utilizes a site-specific recombinase, whereby a region of interest is flanked by two unique 34-bp sequences, known as loxP sites. Expression of the cre protein catalyses recombination between the two loxP sites allowing for translocation, inversion or deletion of the intervening genomic sequence [1] . Although other recombinase systems are available, cre- loxP is the most widely used approach to generate conditional, targeted mutations. The need for a well-characterized, diverse set of cre driver lines is critical, given the enormous investment by the scientific community in the International Knockout Mouse Consortium (IKMC) [2] . This collaborative effort has created an embryonic stem cell library of targeted mutations of nearly all genes in the mouse genome, the majority of which are conditionally targeted using cre- loxP technology. Many cre driver strains, however, display characteristics that were not obvious on their initial generation. Although appreciated anecdotally in individual labs, a few recent publications have highlighted some of these issues in general [3] , [4] . One example is mosaic and/or inconsistent deletion activity, which is seen in Tg(MMTV-cre)4Mam [5] , Krt19 tm1(cre)Mmt (ref. 6 ), Gata4 tm1(cre)Svs (ref. 7 ) and Tg(Nes-cre)1Kln [8] . As many investigators use cre- loxP technology to avoid embryonic lethality associated with traditional knockout schemes, unpredicted activity could pose serious problems if the targeted gene is essential for viability. In addition, unexpected expression, whereby the promoter driving the cre line targets a number of tissues unbeknownst to the designer and user, can lead to misinterpretation of a resulting phenotype. Consistency and precision of the excision activity of a particular cre line is critical for interpretation of experimental results, and will have a major impact on the number of animals that need to be examined before a conclusion is drawn. Examples of this issue can be found for several cre lines, including Tg(Myhc-cre)2182Mds, Osr2 tm2(cre)Jian , Tg(Vil-cre)20Syr and Tg(Ddx4-cre)Idcas, although it is clear this is only a small sample of the frequency of this problem [9] , [10] , [11] , [12] . Interestingly, the parent-of-origin delivering the cre line appears to affect the deletion phenotype, likely due to cre expression in the germ line that persists in the early embryo [13] , [14] , [15] , [16] . Finally, the potential for cre toxicity needs to be addressed given recent findings [17] , [18] . Together, these examples demonstrate that despite the power and versatility of cre driver lines, all of these potential caveats need to be explored systematically to maximize the value of cre resources for the scientific community. We have developed and implemented a pipeline to generate and disseminate detailed information about cre recombinase activity for individual cre driver lines in the JAX Cre Repository (currently 365 strains). Our pipeline identifies cre-mediated recombination at four time points (E10.5, E15.5, P7 and P56) in a wide range of organs, tissues and cell types. The data are permanently archived at the Mouse Genome Informatics CrePortal ( http://www.creportal.org ) and will be updated continuously as work progresses. This study highlights our characterization pipeline and identifies several potentially problematic issues with current cre driver strains that must be considered when designing an experiment using specific strains. On investigation of 40 cre strains, we have found a number of issues with cre function, including unexpected activity in off-target tissues, inconsistent recombination between littermates and differential activity depending on the parent-of-origin of the cre allele. All these factors must be taken into account when choosing a cre driver strain for conditional knockout experiments. Development of the cre characterization pipeline The utility of existing cre driver strains critically depends on careful characterization of their function. Characterization data for most cre strains available in public repositories are limited to that provided by the donating investigators, which is often focused on a specific tissue of interest to their research question. Thus, complementing this data with a standardized characterization pipeline maximizes the value of these resources for the scientific community. We have developed and validated cre reporter assays consisting of standardized protocols, tissues and structures to be assayed, as well as data acquisition and dissemination workflows to streamline the characterization process. To evaluate the functionality of a given cre line, we first considered the most suitable reporter line for use in our pipeline. As our conclusions about the performance of a given cre driver line are based on the expression of a reporter gene, it was essential to choose a reporter line that is ubiquitously expressed following cre excision in all tissues and at all time points. We also considered the robustness of the reporter gene’s expression, which strongly influences the type of detection and imaging technology required for a high-throughput characterization scheme. Finally, breeding performance and availability are additional practical considerations critical for the scalability of the pipeline. We evaluated several reporter lines currently housed as live colonies at The Jackson Laboratory by generating a germline deleted version of each strain. Expression would thus depend entirely on the putatively ubiquitous promoter. 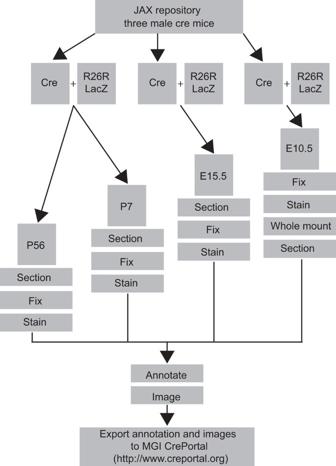Figure 1: Cre strain characterization pipeline used by The Jackson Laboratory Cre Repository. Overview of the pipeline for characterizing new and existing cre driver lines donated to The Jackson Laboratory. Three cre-expressing males are mated to R26R-lacZ reporter females. Litters from one cross are utilized for P56 and P7 time points, whereas timed matings are performed concurrently for embryonic time points, E10.5 and E15.5. P56, P7 and E15.5 litters are necropsied, tissues or embryos frozen, sectioned, stained, imaged and reporter expression is annotated. E10.5 litters are fixed, stained, imaged, sectioned, and reporter expression is annotated. Finally, annotated images are exported to Mouse Genome Informatics (MGI) CrePortal and The Jackson Laboratory’s Cre Repository webpage. The lines examined and critical features are summarized in Table 1 . According to our studies and present needs, the Gt(ROSA)26Sor tm1Sor lacZ (R26R-lacZ) reporter displays a good balance of advantages without any obvious deficiencies [19] ( Supplementary Fig. S1 ). Other strains that work well in one respect, such as robust activity in the case of Tg(CAG-Bgeo/GFP)21Lbe (Z/EG), show deficiencies in other areas, like breeding performance and uniformity of expression domain [20] . It is interesting to note that some Gt(ROSA)26 -targeted reporters display ubiquitous expression and breed well, although the expression level is moderately low when driven using the original splice acceptor scheme. This is not an issue for LacZ, but makes visualization of fluorescent reporters in thin sections difficult. As an additional positive control to authenticate R26R-lacZ reporter results, a small subset of cre strains were crossed to Gt(ROSA)26Sor tm14(CAG-tdTomato)Hze (Rosa-CAG-tdTomato) to ensure that reporter gene expression patterns were consistent ( Supplementary Fig. S2 ). Finally, one advantage to β-galactosidase (β-gal) staining is the ease at which slides can be imaged and permanently archived. Given these considerations, we have chosen to develop our cre characterization pipeline using the R26R-lacZ reporter strain. Table 1 Summary of reporter validation and optimization studies. Full size table The specific ages were chosen to build a streamlined characterization protocol and to generate data that would be useful to the widest range of users. Four time points are used: E10.5, E15.5, postnatal day 7 (P7) and P56. These stages were chosen to capture both developmental and postnatal functionality. A full necropsy is performed at P7 and P56 to isolate a set of 30 individual organs, whereas whole embryos are processed E10.5 and E15.5. After testing of various fixation and processing techniques, we determined that a fresh-frozen/cryosection approach to the E15.5, P7 and P56 time points provided the most robust and reliable signal. For E10.5 embryos, we used a standard whole-mount approach that allowed complete penetration of the X-gal substrate [21] . We have performed a series of control experiments to determine the extent of endogenous activity in our system, which appears to be limited to a few discrete locations in P7 and adult samples ( Supplementary Fig. S3 ). In all cases, multiple specimens from at least two individual litters are analysed, to account for the possibility of individual sample variation. Workflow proceeds by mating multiple male cre mice to female R26R-lacZ reporter mice to produce progeny that will be aged to 8 weeks ( Fig. 1 ). This breeding arrangement is based on both published data and our own experience that a number of cre driver strains display widespread activity when the cre allele is inherited maternally, presumably due to residual pre-zygotic expression of cre [13] , [14] . A second litter from each breeding unit is then taken for the P7 time point, after which timed matings are used to generate E10.5 and E15.5 embryos. Therefore, the entire process can be completed in a total of 12–15 weeks. Figure 1: Cre strain characterization pipeline used by The Jackson Laboratory Cre Repository. Overview of the pipeline for characterizing new and existing cre driver lines donated to The Jackson Laboratory. Three cre-expressing males are mated to R26R-lacZ reporter females. Litters from one cross are utilized for P56 and P7 time points, whereas timed matings are performed concurrently for embryonic time points, E10.5 and E15.5. P56, P7 and E15.5 litters are necropsied, tissues or embryos frozen, sectioned, stained, imaged and reporter expression is annotated. E10.5 litters are fixed, stained, imaged, sectioned, and reporter expression is annotated. Finally, annotated images are exported to Mouse Genome Informatics (MGI) CrePortal and The Jackson Laboratory’s Cre Repository webpage. Full size image After processing, slides are examined and scored for an established set of structures and landmarks. For the adult and P7 time points, this includes a total of 12 broad organ systems, 30 individual organs/structures and 89 substructures ( Supplementary Table S1 ), all of which conform to the proper mouse Anatomical Dictionary (AD) terms to facilitate entry into searchable databases such as CrePortal ( http://www.creportal.org ). For embryonic time points, 13 broad organ systems, 29 individual organs/structures and 73 substructures are annotated using terms conforming to the Mouse Embryo Anatomy Nomenclature Database ( http://emouseatlas.org ; Supplementary Table S2 for E15.5 and Supplementary Table S3 for E10.5). In a few cases, individual cell types are annotated that are not captured by these ontologies, but are likely to be of interest to investigators. Images of slides containing positive staining are captured using the Hamamatsu NanoZoomer 2.0HT digital slide scanning system at X20 magnification. Images of individual annotated organs are then processed and sent to Mouse Genome Informatics for curation into the CrePortal database. 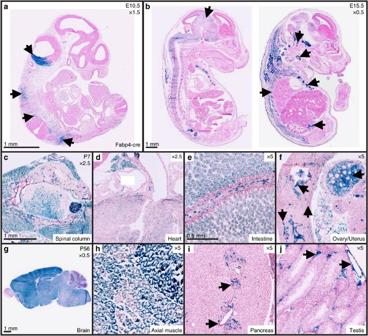Figure 2: Fabp4-cre is widely expressed prenatally and postnatally. (a–j) Cre-mediated β-gal reporter expression showing cre recombination outside white and brown adipose tissue in Fabp4-cre/ROSA26 mice. (a) Histological sections at E10.5 showing β-gal reporter expression in the inferior hindbrain (arrow head), trunk mesenchyme (arrowhead), somites (arrowhead), spinal column and developing dorsal root ganglion (arrowhead). (b) Histological sections at E15.5 showing wide ranging cre activity throughout the central nervous system (arrowhead), inner ear (arrowhead), thyroid gland (arrowhead), vertebra (arrowhead), ribs (arrowhead) and interstitial cells of the testis (arrowhead). (c–f) Selected tissues of postnatal day 7 (P7) mice displaying β-gal expression throughout the spinal column (c), myocardium (d), epithelial and smooth muscle cells of the gut (e), interstitial cell of the ovary, uterine glandular epithelium, myometrium and endometrial cells of the uterus (f) (arrowheads). (g–j) Selected tissues of Adult (P56) mice exhibiting cre activity throughout the brain (g), skeletal muscle (h), islets of Langerhan’s, pancreatic ducts (i) (arrowhead), interstitial cells of the testis and vascular endothelium (j) (arrowhead). As of September 2012, we have published the characterization data for 40 cre strains on http://www.creportal.org ( Table 2 ). However, this is only a minor portion of the total cre strains in JAX Cre Repository (currently 365 strains), as we initially focused on those that see high rates of use or that have been brought to our attention as possibly having unreported activity. This effort is ongoing, and new data are added to creportal regularly. Table 2 Cre recombinase strains currently submitted to creportal.org (Sept. 2012). Full size table The characterization pipeline highlights both reported and unreported cre expression at several time points in a number of cell types and tissues. For example, initial studies using the Tg(Fabp4-cre)1Rev (Fabp4-cre) strain reported abundant expression in adult white and brown adipose tissue with minimal expression in other tissues [22] . Yet, our pipeline analysis indicated expression of the transgene during early organogenesis (E10.5) in developing central nervous system (CNS) structures and trunk mesenchyme ( Fig. 2a ). In concordance with the recent mouse embryo global transcriptome atlas [23] , our data also indicate that Fabp4-cre is expressed in tissues other than adipose during late gestation, such as CNS, glandular tissue, axial bone and testis ( Fig. 2b ). Finally, postnatal expression of the transgene was also shown to be outside of adipose tissue. P7 reporter mice display β-gal activity throughout the spinal cord, dorsal root ganglion, axial muscle ( Fig. 2c ), as well as in the myocardium, intestine, ovary and uterus ( Fig. 2d–f ). P56 mice display similar expression patterns as P7 mice with β-gal being expressed in the CNS, axial muscle and testis, in addition to expression in pancreatic cells (islets of Langerhans and pancreatic ducts; Fig. 2g–j ). Figure 2: Fabp4-cre is widely expressed prenatally and postnatally. ( a – j ) Cre-mediated β-gal reporter expression showing cre recombination outside white and brown adipose tissue in Fabp4-cre/ROSA26 mice. ( a ) Histological sections at E10.5 showing β-gal reporter expression in the inferior hindbrain (arrow head), trunk mesenchyme (arrowhead), somites (arrowhead), spinal column and developing dorsal root ganglion (arrowhead). ( b ) Histological sections at E15.5 showing wide ranging cre activity throughout the central nervous system (arrowhead), inner ear (arrowhead), thyroid gland (arrowhead), vertebra (arrowhead), ribs (arrowhead) and interstitial cells of the testis (arrowhead). ( c – f ) Selected tissues of postnatal day 7 (P7) mice displaying β-gal expression throughout the spinal column ( c ), myocardium ( d ), epithelial and smooth muscle cells of the gut ( e ), interstitial cell of the ovary, uterine glandular epithelium, myometrium and endometrial cells of the uterus ( f ) (arrowheads). ( g – j ) Selected tissues of Adult (P56) mice exhibiting cre activity throughout the brain ( g ), skeletal muscle ( h ), islets of Langerhan’s, pancreatic ducts ( i ) (arrowhead), interstitial cells of the testis and vascular endothelium ( j ) (arrowhead). Full size image Unreported or unexpected cre activity in off-target tissues One of the most striking findings apparent in a number of cre strains was the frequency of unreported/unexpected deletion activity. 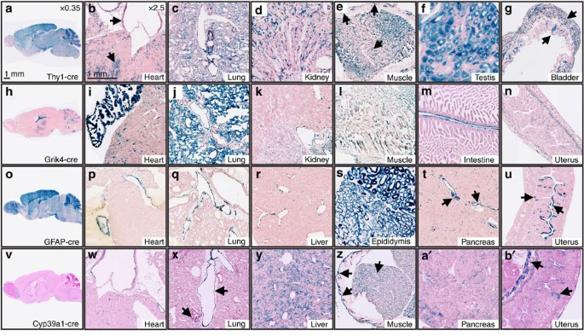Figure 3: Recombination in ‘off-target’ tissues of neural-specific cre driver lines. (a,b′) Select adult (P56) tissue sections indicating off target recombination in several neural-specific cre lines after crossing to the R26R-lacZ reporter line. (a,h,o,v) Cre-mediated β-gal expression in Thy1-cre (a), Grik4-cre (h), GFAP-cre (o) and Cyp39a1-cre (v) target tissues (brain). (b–g) Additional cre activity in Thy1-cre mice is present in the myocardium and vascular endothelium (b), lung tissue (arrowheads) (c), renal tubules (d), skeletal muscle, hair follicles, skin (arrowheads) (e), seminiferous tubules (f) and smooth muscle and urothelial cells of the bladder (arrowheads) (g). (i–n) Off-target cre activity in Grik4-cre mice is observed in the myocardium (i), lung tissue (j), renal tubules (k), skeletal muscle (l), smooth muscle cells of the intestine (m) and myometrium (n). (p–u) Observed off-target cre recombinase expression in Gfap-cre mice occurs in the endocardium (p), pulmonary vascular endothelium (q), endothelial cells of the liver portal system (r), ductus epididymis (s), islets of Langerhan’s and pancreatic duct endothelium (arrowheads) (t), as well as endometrial and glandular endometrial cells of the uterus (arrowheads) (u). (w–b′) Unreported cre recombination is present in several tissues of the Cyp39a1-cre mouse including the myocardium, aortic endothelial cells (w), pulmonary vascular endothelium and bronchiolar epithelial cells (arrowheads) (x), hepatocytes (y), skeletal muscle, hair follicles, skin (arrowheads) (z), acinar cells (a′) and uterine smooth muscle cells and endometrium (arrowheads) (b′). Figure 3 shows several examples that range from restricted deletion outside of the target tissue to widespread activity in nearly all tissue types. Tg(Thy1-cre)1Vln (Thy1-cre) was initially generated to express cre recombinase in postnatal cortex and hippocampal neurons [24] . Although Thy1-cre is expressed robustly throughout postnatal brain it is also widespread throughout many additional tissues ( Fig. 3a ). We detected reporter expression throughout the myocardium, vascular endothelium, lung alveoli and bronchiole cells, renal tubules, skeletal muscle, skin, hair follicles, testis and bladder ( Fig. 3b–g ). Tg(Grik4-cre)G32-4Stl (Grik4-cre) has been reported to be active in the CA3 region of the hippocampus by E13.5 with low cre recombination rates in other parts of the brain [25] . We observe hippocampal expression ( Fig. 3h ), as well as widespread activity in heart and lung tissue ( Fig. 3i ), with more restricted patterns in renal tubules, skeletal muscle, smooth muscle of the intestine and myometrium ( Fig. 3k–n ). The Tg(GFAP-cre)25Mes (GFAP-cre) strain under control of the human glial fibrillary acidic protein promoter was reported to primarily target CNS glia, but some recombination occurs in periportal cells of the liver [26] . Figure 3o shows staining in adult brain, displaying homogenous expression of β-gal in all cells of the olfactory bulb, cortex and cerebellum, with mosaic expression, the result of a mixed population of β-gal positive and negative cells, throughout remaining structures. In addition to periportal cells, we observe varying levels of recombination in several other tissues including endocardium, pulmonary vascular endothelium, epididymis, islets of Langerhans, pancreatic ducts, endometrium and glandular endometrium ( Fig. 3p–u ) [26] . Finally, Tg(Cyp39a1-cre)1Aibs (Cyp39a1-cre) was generated to target various CNS structures, but no other tissue was assayed for cre expression ( Fig. 3v ). Our pipeline identified abundant, wide-ranging reporter expression in the myocardium, vascular endothelium, bronchioles, hepatocytes, skeletal muscle, hair follicles, skin, pancreatic acinar cells, uterine smooth muscle and endometrium ( Fig. 3w–b′ ) It is important to note that not all unreported and/or unexpected activity is due to ectopic expression of the cre transgene, but is potentially also due to proper, but unappreciated, expression of the driver gene itself. In addition, because most transgenic cre driver strains are made with discrete pieces of the proximal promoter of a given gene, the limited complement of enhancers and repressors might permit more widespread expression. Integration site effects are also likely to influence transgene expression patterns. Figure 3: Recombination in ‘off-target’ tissues of neural-specific cre driver lines. ( a , b′ ) Select adult (P56) tissue sections indicating off target recombination in several neural-specific cre lines after crossing to the R26R-lacZ reporter line. ( a , h , o , v ) Cre-mediated β-gal expression in Thy1-cre ( a ), Grik4-cre ( h ), GFAP-cre ( o ) and Cyp39a1-cre ( v ) target tissues (brain). ( b – g ) Additional cre activity in Thy1-cre mice is present in the myocardium and vascular endothelium ( b ), lung tissue (arrowheads) ( c ), renal tubules ( d ), skeletal muscle, hair follicles, skin (arrowheads) ( e ), seminiferous tubules ( f ) and smooth muscle and urothelial cells of the bladder (arrowheads) ( g ). ( i – n ) Off-target cre activity in Grik4-cre mice is observed in the myocardium ( i ), lung tissue ( j ), renal tubules ( k ), skeletal muscle ( l ), smooth muscle cells of the intestine ( m ) and myometrium ( n ). ( p – u ) Observed off-target cre recombinase expression in Gfap-cre mice occurs in the endocardium ( p ), pulmonary vascular endothelium ( q ), endothelial cells of the liver portal system ( r ), ductus epididymis ( s ), islets of Langerhan’s and pancreatic duct endothelium (arrowheads) ( t ), as well as endometrial and glandular endometrial cells of the uterus (arrowheads) ( u ). ( w – b′ ) Unreported cre recombination is present in several tissues of the Cyp39a1-cre mouse including the myocardium, aortic endothelial cells ( w ), pulmonary vascular endothelium and bronchiolar epithelial cells (arrowheads) ( x ), hepatocytes ( y ), skeletal muscle, hair follicles, skin (arrowheads) ( z ), acinar cells ( a′ ) and uterine smooth muscle cells and endometrium (arrowheads) ( b′ ). Full size image Maternal versus paternal inheritance of the cre transgene Interestingly, the parent-of-origin of the cre transgene can be an important consideration when planning experimental strategies. Maternal inheritance of the cre transgene has been shown to affect cre excision patterns [9] . This is likely due to post-zygotic persistence of the cre protein expressed from the female germline. Examples include the Tg(Ddx4-cre)1Dcas (Vasa-cre) [13] and Tg(Sox2-cre)1Amc (Sox2-cre) lines [27] . Our data indicate that Tg(EIIa-cre)C5379Lmgd (EIIa-cre) may also variably express cre depending on the parental inheritance of the transgene. 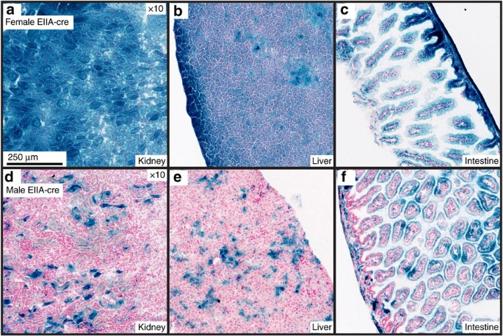Figure 4: Parent-of-origin affects recombination of EIIa-cre in vivo. (a–f) Histological sections showing cre-mediated β-gal activity in select tissues from pups that inherited the EIIa-cre transgene either maternally (a–c) or paternally (d–f). Figure 4 highlights the differences in cre recombination in select tissues when the EIIa-cre transgene is inherited through the maternal ( Fig. 4a–c ) or paternal ( Fig. 4d–f ) germline. Offspring inheriting EIIa-cre maternally exhibit widespread reporter expression in all assayed tissues, such as the kidney ( Fig. 4a ), liver ( Fig. 4b ), gut, ( Fig. 4c ) and pancreas, except the spleen that exhibited mosaic labelling (data not shown). Paternally inherited EIIa-cre promotes mosaic recombination throughout all tissue analysed, including the kidney ( Fig. 4d ), liver ( Fig. 4e ), gut ( Fig. 4f ), spleen, pancreas, heart, lung, muscle and thymus (data not shown). Figure 4: Parent-of-origin affects recombination of EIIa-cre in vivo. ( a – f ) Histological sections showing cre-mediated β-gal activity in select tissues from pups that inherited the EIIa-cre transgene either maternally ( a – c ) or paternally ( d – f ). Full size image Inconsistent cre recombination between littermates Consistency in cre activity is also critically important for accurate interpretation of experimental results. Variability in cre activity can result from poor expression, which leads to inconsistent mosaicism in target tissues. We have also observed more marked examples of inconsistent activity, wherein cre excision varies from tissue specific to ubiquitous within a single litter [9] , such as Tg(Tek-cre)12Flv (Tek-cre) and Tg(Vav1-cre)A2Kio (Vav1-cre). Tek-cre was generated using the promoter/enhancer sequences of the endothelial-specific tyrosine kinase ( Tek / TIE2 ). Previous work localized cre recombination to endothelial cells, hematopoietic cells and their precursors allowing for endothelial cell fate mapping as well as conditional gene targeting in this cell compartment [28] , [29] , [30] . However, we observed that litters generated by crossing R26R-lacZ females to Tek-cre males can yield inconsistent cre recombination. As shown in Fig. 5a , E10.5 embryos from the same litter display very different levels of cre excision, ranging from endothelial-specific ( Fig. 5a ) to nearly ubiquitous in non-target tissues ( Fig. 5b ). We also saw a similar effect in Vav1-cre mice, for which cre recombination has been reported in hematopoietic cells [31] , [32] . Littermates of R26R-lacZ/Vav1-cre crosses exhibit variable cre activity. E10.5 embryos display restricted reporter expression in the hepatic primordium ( Fig. 5c ) or mosaic expression throughout the embryo ( Fig. 5d ). It is important to note that inconsistencies in reporter gene expression were ruled out by reproducing the same expression patterns using a CAG-driven fluorescent reporter ( Supplementary Fig. S2 ). The above data indicate that unpredictable widespread cre excision can occur in lines that generally exhibit specific recombination patterns. 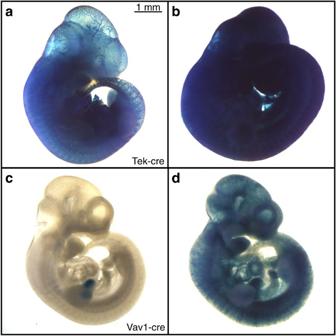Figure 5 Inconsistent cre activity in E10.5 littermates in Tek-cre and Vav1-cre strains.E10.5 embryos collected from timed matings between R26R-lacZ female mice and male mice harbouring the cre allele indicated. (a,b) Tek-cre/R26R-lacZ littermates exhibiting restricted (a) or homogenous and (b) β-gal expression. (c,d) Vav1-cre/R26R-lacZ littermates displaying β-gal restricted to hepatic primordium (c) or mosaic expression throughout embryo (d). Figure 5 Inconsistent cre activity in E10.5 littermates in Tek-cre and Vav1-cre strains. E10.5 embryos collected from timed matings between R26R-lacZ female mice and male mice harbouring the cre allele indicated. ( a , b ) Tek-cre/R26R-lacZ littermates exhibiting restricted ( a ) or homogenous and ( b ) β-gal expression. ( c , d ) Vav1-cre/R26R-lacZ littermates displaying β-gal restricted to hepatic primordium ( c ) or mosaic expression throughout embryo ( d ). Full size image The cre- loxP system has arguably become the standard method for generating conditional null alleles [33] , [34] , [35] . Here, we report a high-throughput scheme for the extensive characterization of cre excision activity in driver lines that ends in the dissemination of valuable data to the research community via a publicly accessible database. We also illustrate several issues that must be taken into account when using cre driver lines. For example, several cre strains, specifically neuro-specific strains, exhibited significant unexpected and unreported deletion outside of their targeted tissue or cell types. We also show that cre activity can vary based on maternal or paternal inheritance of the allele and that inconsistent recombination between littermates was also observed. The development of a system for analysing cre activity in driver lines should take into account sensitivity, throughput, comprehensiveness and data dissemination. After extensive testing of several cre reporter strain options ( Table 1 ), we settled on the R26R-lacZ strain [19] , [36] because it provided the most robust, reliable and ubiquitous reporter expression. R26R-lacZ mice exhibit a very minor level of background signal, induced by endogenous mammalian β-gal in a small subset of tissues ( Supplementary Fig. S3 ), which is easily distinguished from authentic reporter expression. R26R-lacZ mice are appropriate tools for creating a sensitive and high-throughput cre characterization system. Enzymatic reporters offer a high degree of sensitivity by amplifying the visible signal created by cre excision. Although paraffin section immunohistochemistry could be utilized with reporters to obtain better cellular morphology; we found β-gal staining of fresh-frozen cryosections gave a higher level of sensitivity in assaying cre activity. Furthermore, β-gal staining protocols are amenable to both high-throughput batch procedures and permanent archiving of slides, in contrast to fluorescent-based cre reporters. The ages and tissues chosen for analysis were based on building a thorough streamlined characterization protocol, and generating data that would be useful to the widest range of users. Standardization of tissue and structure annotation criteria at E10.5, E15.5, P7 and P56, in accordance with defined vocabularies from the Embryonic Mouse AD [37] and Adult Mouse AD [38] , facilitates the integration of data with searchable databases, such as CrePortal. A realistically comprehensive characterization of cre excision is obtained by assaying activity in a broad range of organ systems, substructures and cell types at varied time points. Recognizing that no characterization scheme will be totally comprehensive, our approach seeks to balance the need for reasonable throughput with the goal of maximizing the characterization of informative tissues and time points. Both the granularity of this characterization and the consistency of annotation with anatomical dictionaries increase the utility of the data for the research community. To maximize the utility of the cre characterization resource, all data described above were made publicly available to the scientific community via CrePortal ( http://www.creportal.org ). For each cre strain, we link a specific organ/tissue annotation to coordinates on the appropriate slide scan. This format allows the user to zoom and move around the slide as desired, viewing all characterization data directly and interactively. This approach greatly reduces the time required to generate and upload the images to the CrePortal database, while giving the user a comprehensive view of histological cre characterization data. Through this web resource, investigators will save time and effort in determining appropriate cre lines for their experimental needs, be able to view and compare cre activity data and link directly to the repositories distributing cre mice. Resources such as CrePortal will become increasingly important as the use of IKMC conditional alleles accelerates. One of the most common observations with cre lines examined thus far is unexpected/unreported cre expression. In some cases, these off-target effects are reported, but for the most part the published literature focuses on the performance of the cre line in the specific target tissue and other tissues are rarely examined [9] , [10] , [11] , [12] . The lines highlighted here, Thy1-cre, Grik4-cre, GFAP-cre and Cyp39a1-cre, were created using transgenic approaches, and as such the observed unexpected activity could result from integration site-mediated alteration of expression patterns, differences in copy number or epigenetic alteration of the transgene. [3] Although a knock-in approach could, in theory, circumvent such issues, specificity problems can occur with both designs when unexpected expression is a result of endogenous or ectopic gene activity. For example, Foxg1 tm1(cre)Skm ( Foxg1 -cre) was created as a targeted mutation, yet displays varying levels of unexpected cre activity dependent on strain background. [39] Such effects are likely due to endogenous Foxg1 activity that is partially altered by background-specific modifiers. Interestingly, recent studies have also highlighted phenotypic effects of haploinsufficiency in this same cre strain, indicating another caveat to be considered when choosing cre strains generated via targeted mutation [40] . It is likely that some of the cases of unforeseen cre activity shown here were a result of natural developmental and physiological roles of the gene promoter driving cre expression. As cre marks cell lineages, brief bursts of expression early in development can have a profound effect on the extent of excision at later stages. Furthermore, unexpected recombination in the germline can cause sporadic ubiquitous deletion as F1 mice are bred to obtain animals hemizygous for cre and homozygous for the floxed allele [12] . Although for some experiments unanticipated activation might be acceptable (for example, those looking to simply bypass embryonic lethality), any experiment designed to establish cell autonomy of gene function could be compromised if off-target effects are not accounted for, or if cre strain functionality is not properly specific. In addition to unreported, off-target cre activity, parent-of-origin effects on cre excision can confound experimental results. In the example shown, EIIa-cre maternal inheritance resulted in uniform deletion, whereas paternal inheritance showed mosaic expression in the same tissues. It has been previously reported that EIIa-cre males yield a proportion of progeny exhibiting mosaic cre deletion patterns [41] . In the female germline, the EIIa promoter directs cre activity to the unfertilized egg, whereas in the male germline, cre is not expressed until after fertilization occurs [41] , [42] . Such mosaic deletion is typically circumvented by the practice of breeding a subsequent generation, thereby relying on germline deletion of the floxed allele. However, B6.EIIA-cre is a line also utilized to attempt full somatic deletion in a single generation. Experiments using F1 progeny from such a deleter cross would be widely variable depending on whether the cre allele was transmitted by the male or female parent. Accordingly, EIIa-cre provides an interesting and useful example of how maternal versus paternal cre inheritance can affect excision efficiency and thus experimental design. Although less common, male germline deletion in other strains has also been reported [43] , emphasizing the importance of careful characterization of cre strains before use in experiments. Inconsistent cre excision within a single experimental litter carries the risk of complicating phenotypic analyses and potentially re-introducing the embryonic lethality that conditional knockout strategies aim to avoid. Examples reported here, Tek-cre and Vav1-cre, show sporadic ubiquitous deletion. It is likely that such ubiquitous excision is a result of germline effects, or variable precocious cre expression in very early embryogenesis [9] . Regardless of mechanism, such activity can confound phenotypic analysis, particularly in case where questions of cell autonomy are being addressed. Despite advances in the development of tissue- and cell-specific cre driver lines, data shown here illustrate that the fidelity of cre activity is often not ideal [4] , [10] . A number of mechanisms could potentially explain these observations, including transgene insertion site activation or silencing, undocumented gene expression patterns, incomplete incorporation of regulatory elements into the driver construct, modification by strain genetic background, transgene silencing/copy number changes and maternal/paternal germline expression. Moreover, unexpected excision largely goes unreported, and as a cre line becomes adopted as a common tool, it is essential that users be aware of the full range of potential cre activity. Current large-scale mouse gene targeting projects, such as IKMC, will generate an incredibly valuable set of loxP -flanked alleles to the scientific community [2] . However, proper utilization of these resources will only be realized with a set of well-characterized cre-driver lines. Thus, complementing the published data with a standardized, unbiased and extensive characterization pipeline promises to maximize the value of these tools for the scientific community. Mice All strains used in this study were obtained from The Jackson Laboratory. Specific cre lines are listed in Table 2 . The following reporter strains were used in this study: B6.129S4- Gt(ROSA)26Sor tm1Sor /J (R26R-lacZ, JAX stock no. 003474) [19] , B6;129- Gt(ROSA)26Sor tm2Sho /J (R26R-GFP, JAX stock no. 004077) [44] , B6.129 × 1- Gt(ROSA)26Sor tm1(EYFP)Cos /J (R26R-YFP, JAX stock no. 006148) [45] , B6.129(Cg)-Tg(CAG-Bgeo/GFP)21Lbe/J (Z/EG, JAX stock no. 004178) [20] , B6.Cg-Tg(CAG-Bgeo, -DsRed*MST)1Nagy/J (DsRed, JAX stock no. 006055) [45] , STOCK Gt(ROSA)26Sor tm4(ACTB-tdTomato, -EGFP)Luo /J (mT/mG, JAX stock no. 007576) [46] and B6.Cg- Gt(ROSA)26Sor tm14(CAG-tdTomato)Hze /J (Rosa-CAG-tdTomato, JAX stock no. 007914) [47] . Males from the indicated cre driver lines were bred to female R26R-lacZ reporters, except for maternal inheritance experiments involving EIIa-cre mice. For postnatal time points (P7 and P56), mice were housed in permanent trio matings. Timed trio matings for embryonic day 10.5 (E10.5) and embryonic day 15.5 (E15.5) were set in the evening, and checked for the appearance of a vaginal plug the following morning. The appearance of a vaginal plug was denoted as embryonic day 0.5. All procedures were approved by The Jackson Laboratory’s Institutional Animal Care and Use Committee and performed in accordance with the National Institutes of Health guidelines for the care and use of animals in research. Genotyping Embryos, pups and adult mice were genotyped for the presence of cre by amplification of DNA extracted from yolk sacks, embryonic limbs or tail tips, respectively. The following generic cre PCR primers were used to amplify a 600-bp fragment of genomic DNA: crefwd 5′-CATTTGGGCCAGCTAAACAT-3′ and crerev 5′-CAGACCAGGCCAGGTATCTC-3′. Tissue collection P56 mice and pregnant dams were euthanized by CO 2 asphyxiation, whereas P7 pups were decapitated. P56 and P7 tissues ( Supplementary Table S1 ) were dissected and immediately frozen in Tissue-Tek optimal cutting temperature (Sakura Finetek, Torrance, CA, USA) on dry ice. Following CO 2 asphyxiation of pregnant females, embryos were immediately dissected from extra-embryonic tissues in ice-cold 1 × phosphate-buffered saline (PBS). E15.5 embryos were immediately frozen in optimal cutting temperature on dry ice. Frozen tissues and embryos were stored at −20 °C until cryosectioning. E10.5 embryos were fixed on ice with 0.2% glutaraldehyde (Electron Microscopy Sciences; Hatfield, PA, USA) in 0.1 M phosphate buffer (pH 7.3) with 5 mM EGTA and 2 mM MgCl 2 and stained immediately. For experiments utilizing Rosa-CAG-tdTomato reporters, E10.5 embryos were fixed in 4% paraformaldehyde in 1 × PBS at 4 °C, washed in 3 × 15 min in 1 × PBS and imaged in whole mount to visualize fluorescence. Histology and β-gal staining β-Gal staining of fresh-frozen cryosections and whole-mount embryos was performed as described previously [21] , [48] . Specific details of the β-gal assay used for this study are briefly described below. Detailed protocols are available on our website, http://cre.jax.org . Frozen sections Ten micrometre cryosections of all P7 and P56 tissues and whole E15.5 embryos were placed onto Superfrost Plus slides (Fisher Scientific; Pittsburgh, PA, USA) and stored at −80 °C until staining. Sections were fixed in 0.2% glutaraldehyde in 1 × PBS on ice for 10 min, washed in 1 × PBS and then washed in detergent rinse (0.1 M phosphate buffer (pH 7.4) with 2 mM MgCl 2 , 0.02% Igepal (Sigma; St Louis, MO, USA) and 0.01% sodium deoxycholate) for 10 min. For β-gal staining, slides were incubated overnight at 37 °C fully immersed in a solution of 1 mg ml −1 5-bromo-4-chloro-3-indolyl-β- D -galactopyranoside (X-gal; AppliChem; Darmstadt, Germany) staining solution (0.1 M phosphate buffer (pH 7.4) with 2 mM MgCl 2 , 0.02% Igepal, 0.01% sodium deoxycholate, 5 mM potassium ferricyanide and 5 mM potassium ferrocyanide). Following staining, slides were post-fixed in 4% paraformaldehyde in 1 × PBS, counterstained with Nuclear Fast Red (Vector Laboratories; Burlingame, CA, USA), dehydrated through a series of ethanol, ethanol/xylenes and xylene washes (Fisher Scientific; Fairlawn, NJ, USA) and mounted with Permount (Fisher Scientific). Whole-mount embryos Following fixation, E10.5 embryos were washed and permeabilized in detergent rinse and incubated overnight at 37 °C in 1 mg ml −1 X-gal staining solution. Embryos were then post-fixed in 4% paraformaldehyde in PBS at 4 °C overnight, and cleared in 50% glycerol before whole-mount imaging (see below) and embedding. Finally, stained embryos were embedded in paraffin, sectioned at 5 μm onto Superfrost Plus slides, counterstained with Nuclear Fast Red and mounted with Permount. Imaging X-gal-stained embryos and Rosa-CAG-tdTomato × cre embryos were imaged in whole mount using a Leica MZ16 FA fluorescence stereoscope equipped with a DFC 490 camera and Planapo × 1.0 objective (Leica: Wetzlar, Germany). For imaging fluorescence, a Leica EL6000 excitation source was used in conjunction with a DsRed appropriate filter cube (Leica DSR, 545/30 excitation filter; Leica). X-gal-stained slides were scanned at X20 magnification using a NanoZoomer 2.0-HT slide scanner (Hamamatsu). How to cite this article: Heffner, C. S. et al. Supporting conditional mouse mutagenesis with a comprehensive cre characterization resource. Nat. Commun. 3:1218 doi: 10.1038/ncomms2186 (2012).